Molecular insights into the membrane-associated phosphatidylinositol 4-kinase IIα Phosphatidylinositol 4-kinase IIα (PI4KIIα), a membrane-associated PI kinase, plays a central role in cell signalling and trafficking. Its kinase activity critically depends on palmitoylation of its cysteine-rich motif (-CCPCC-) and is modulated by the membrane environment. Lack of atomic structure impairs our understanding of the mechanism regulating kinase activity. Here we present the crystal structure of human PI4KIIα in ADP-bound form. The structure identifies the nucleotide-binding pocket that differs notably from that found in PI3Ks. Two structural insertions, a palmitoylation insertion and an RK-rich insertion, endow PI4KIIα with the ‘integral’ membrane-binding feature. Molecular dynamics simulations, biochemical and mutagenesis studies reveal that the palmitoylation insertion, containing an amphipathic helix, contributes to the PI-binding pocket and anchors PI4KIIα to the membrane, suggesting that fluctuation of the palmitoylation insertion affects PI4KIIα’s activity. We conclude from our results that PI4KIIα’s activity is regulated indirectly through changes in the membrane environment. Phosphatidylinositol 4-kinase IIα (PI4KIIα), the most abundant PI4K in mammalian cells and mainly localized in the trans-Golgi network (TGN) and endosomes [1] , [2] , produces more than half of the Golgi phosphatidylinositol 4-phosphate (PI4P) and is involved in many different cell pathways including PI(4,5)P 2 synthesis, membrane trafficking (regulating endosomal sorting of signalling receptors and promoting adaptor protein recruitment to endosomes and TGN) [3] , [4] , [5] , signal transduction (Wnt and HER-2 signalling pathways) [6] , [7] , [8] , phagocytosis [9] and the exo–endocytic cycle of synaptic vesicles [10] . Its dysfunction contributes to tumour growth [6] , spastic paraplegia [11] , Gaucher’s disease [12] and Alzheimer’s disease [13] , [14] , suggesting PI4KIIα as a drug target. The PI4K family includes type II PI4Ks (PI4KIIα and PI4KIIβ) and type III PI4Ks (PI4KIIIα and PI4KIIIβ). Unlike PI4KIIIs that belong to the PI 3/4 kinase family and are structurally similar to PI3Ks, PI4KIIs have a catalytic region that differs substantially from the one found in PI3Ks [15] . PI4KIIα is insensitive to inhibitors of PI3Ks, but can be inhibited by ADP, AMP and adenosine [15] , [16] , [17] . Although many specific high-quality isoform-selective inhibitors of PI3Ks have been developed [18] , [19] , [20] based on the crystal structures of PI3Ks [21] , [22] , [23] , [24] and some of them, such as PX866 (ref. 25 ), GS-1101 (ref. 26 ) and PI-103 (refs 18 , 27 ), have already been tested in clinical trials, no specific inhibitor for PI4KIIα is currently available. PI4KIIα has a specific cysteine-rich motif (-CCPCC-); its kinase activity critically depends on palmitoylation of the cysteine-rich motif [15] , [28] , [29] and is modulated by cholesterol, amyloid-β peptide, mastoparan, 25-hydroxycholesterol and ginsenoside (20S)Rg3 via changing the membrane environment as suggested previously [14] , [30] , [31] , [32] . Considering the emerging importance of PI4KIIα in cell signalling and diseases, the availability of structural information on PI4KIIα would not only reveal its substrate specificity and kinase activity regulation, but also could assist in drug development for PI4KIIα-related diseases. In this study, we report the crystal structure of human PI4KIIα catalytic domain in its ADP-bound form at 2.95 Å resolution. Besides the nucleotide-binding pocket differing notably from that found in PI3Ks, two novel structural insertions of PI4KIIα, a palmitoylation insertion and an RK-rich insertion, contribute to its ‘integral’ membrane-binding feature via both hydrophobic and electrostatic interactions. Molecular dynamics (MD) simulations and biochemical studies suggest that changes in membrane dynamics and fluidity modulate the fluctuation of PI4KIIα’s palmitoylation insertion, affecting the conformation of the substrate-binding pocket and, thereby, regulating kinase activity. Overall structure Full-length human PI4KIIα contains a Pro-rich amino-terminal domain (1–93) and a carboxy-terminal catalytic domain (94–479) [33] , the latter including a palmitoylation motif - 174 CCPCC 178 - ( Fig. 1a ). As an integral membrane protein, PI4KIIα is prone to aggregate. 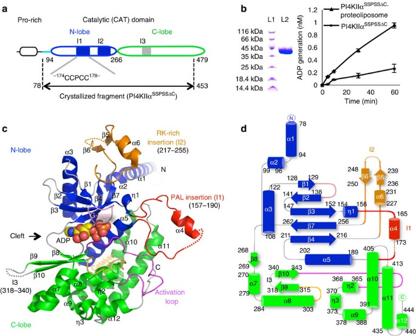Figure 1: Overall structure of the human PI4KIIα catalytic domain. (a) Primary structure of PI4KIIα. I1, I2 and I3 represent three insertions in PI4KIIα not found in PI3Ks. Palmitoylation and RK-rich insertions are referred as I1 and I2, respectively. The crystallized fragment PI4KIIαSSPSSΔCis indicated by a black arrow. (b) Purification and kinase activity assay of PI4KIIαSSPSSΔC. The kinase activity of PI4KIIαSSPSSΔCin PI/Triton X-100 (0.2%)(▴) or PI-containing liposome/Triton X-100 (0.2%)(▪) was measured by monitoring ADP production. The error bars represent the s.d. from three independent experiments. (c) Overall structure of the ADP-bound PI4KIIα catalytic domain. Untraced segments are depicted with dashed lines. The G-loop, catalytic loop and activation loop are coloured in pink, bright orange and magenta, respectively. The palmitoylation insertion (PAL insertion, I1) and RK-rich insertion (I2) are coloured in red and gold, respectively. ADP is shown in a sphere model and is coloured according to its atoms (carbon, yellow; oxygen, red; nitrogen, blue; phosphorus, orange). The colour scheme here is used in all figures unless otherwise mentioned. (d) Secondary structure topology of the PI4KIIα catalytic domain. All structural figures were prepared with PyMol (DeLano, 2002,http://www.pymol.org) or UCSF Chimera (http://www.cgl.ucsf.edu/chimera/). We therefore screened a fragment PI4KIIα SSPSSΔC ( Supplementary Table 1 ), which could be purified to high homogeneity and crystallized into high-quality crystals. Although the purified PI4KIIα SSPSSΔC showed low kinase activity in solution, once it was reconstituted in liposomes, its kinase activity increased approximately fivefold to a level nearly close to that of the wild type ( Fig. 1b ); moreover, this construct still associated with membranes when expressed in E. coli . These observations suggest that PI4KIIα SSPSSΔC preserves the active conformation of the wild-type PI4KIIα catalytic domain. All PI4KIIα constructs (including PI4KIIα SSPSSΔC ) used in the present study are described and summarized in Supplementary Table 1 . Figure 1: Overall structure of the human PI4KIIα catalytic domain. ( a ) Primary structure of PI4KIIα. I1, I2 and I3 represent three insertions in PI4KIIα not found in PI3Ks. Palmitoylation and RK-rich insertions are referred as I1 and I2, respectively. The crystallized fragment PI4KIIα SSPSSΔC is indicated by a black arrow. ( b ) Purification and kinase activity assay of PI4KIIα SSPSSΔC . The kinase activity of PI4KIIα SSPSSΔC in PI/Triton X-100 (0.2%)( ▴ ) or PI-containing liposome/Triton X-100 (0.2%)(▪) was measured by monitoring ADP production. The error bars represent the s.d. from three independent experiments. ( c ) Overall structure of the ADP-bound PI4KIIα catalytic domain. Untraced segments are depicted with dashed lines. The G-loop, catalytic loop and activation loop are coloured in pink, bright orange and magenta, respectively. The palmitoylation insertion (PAL insertion, I1) and RK-rich insertion (I2) are coloured in red and gold, respectively. ADP is shown in a sphere model and is coloured according to its atoms (carbon, yellow; oxygen, red; nitrogen, blue; phosphorus, orange). The colour scheme here is used in all figures unless otherwise mentioned. ( d ) Secondary structure topology of the PI4KIIα catalytic domain. All structural figures were prepared with PyMol (DeLano, 2002, http://www.pymol.org ) or UCSF Chimera ( http://www.cgl.ucsf.edu/chimera/ ). Full size image PI4KIIα SSPSSΔC with ADP-bound formed crystals in the space group I422. The crystal structure was determined at 2.95 Å resolution ( Table 1 ; Fig. 1c,d , Supplementary Fig. 1 ). The resolved structure comprises an N-terminal flexible helix α1 (78–94) and a catalytic domain that is divided into an N-lobe (95–265) and a C-lobe (266–453). The N-lobe contains a five-stranded antiparallel β-sheet core (β1-β2-β3-β7-β4) flanked by a helical hairpin (α2 and α3) on one side and helix α5 on the other. The C-lobe contains the helices α8, η2, η3, α9, α10, α11 and α12, which form a helical bundle together with N-lobe helix α5. The helical bundle is flanked by three β-strands (β8, β9 and β10) and helix α7. Table 1 Data collection and refinement statistics. Full size table There are two molecules (A and B) per asymmetric unit in the crystal. Molecule A and B adopt different orientations of their N-terminal helix α1 ( Supplementary Fig. 2a ). By investigating the crystal packing, we found that molecule A and B, respectively, forms similar octamers (A 8 and B 8 ) with their own crystallography symmetric molecules ( Supplementary Fig. 2b–d ). Although the buried surfaces within octamers are significant according to the analysis by PISA [34] , the oligomerization state of membrane-bound PI4KIIα needs further investigation. Both PI3Ks and PI4KIIα share a common catalytic kinase domain with N-lobe and C-lobe ( Supplementary Fig. 3a ). The root mean square deviation of aligned coordinates between the catalytic domains of PI4KIIα and PI3Kα (p110α, PDB code, 2RD0), PI3Kβ (p110β, PDB code, 2Y3A), PI3Kγ (p110γ, PDB code, 1E8X), PI3Kδ (p110δ, PDB code, 2WXF), Vps34 (PDB code, 2X6H) and PIP4KIIβ (PDB code, 1BO1) are 3.08 Å, 3.18 Å, 3.50 Å, 2.89 Å, 3.60 Å and 3.82 Å, respectively. Besides, the catalytic domain of PI4KIIα has three novel insertions that are not found in PI3Ks, namely I1 and I2 in the N-lobe and I3 in the C-lobe ( Fig. 1c,d ). I1 (157–190) is inserted between helix η1 and α5 and contains an amphipathic α-helix (α4, 165–173, Supplementary Fig. 1b ) followed by the palmitoylation motif - 174 CCPCC 178 -, and hereinafter referred to as the palmitoylation insertion. I2 (217–255), referred to as the RK-rich insertion (contains an abundance of Arg and Lys residues), is inserted between strands β4 and β7 and consists of one helix (α6) and two small β-strands (β5 and β6). I3 (318–340), located between β9 and β10 in the C-lobe, could not be built due to its lack of electron density. Structure-based sequence alignment between PI4KIIα and PI3Ks reveals three loops related to kinase activity, the glycine-rich G-loop (130–136), the catalytic loop (308–315) and the activation loop (344–364) ( Fig. 1c,d , Supplementary Fig. 3 ). The G-loop, which has been reported to bind to the phosphate group of nucleotides [21] , shows no consensus between PI4KIIα and PI3Ks ( Supplementary Fig. 3b ), but is highly conserved among PI4KIIs from different species ( Supplementary Fig. 4 ); being a conserved feature the G-loop should contribute to the nucleotide-binding specificity of PI4KIIs. Interestingly, the closest structural analogues of PI4KIIα found by use of the DALI server [35] are not lipid kinases but protein kinases, including a helicobacter pylori proinflammatory kinase CTKA (PDB code, 3AKK), the Golgi casein kinase (PDB code, 4KQB) and the actin-fragmin kinase (PDB code, 1CJA), which implies an evolutionary relationship between PI4KIIα and protein kinases. It should be noted that the insertions I1, I2 and I3 are unique to PI4KIIα; they also do not arise in the protein kinases’ structural analogues. Nucleotide-binding site The crystal structure of PI4KIIα in the ADP-bound state identifies the nucleotide-binding pocket ( Fig. 2a ). Both Ser134 and Ser137 donate hydrogen bonds that grasp the β-phosphate of ADP. Lys152 and Asp346 hold the α-phosphate in position via a salt bridge and hydrogen bonds, respectively. In addition, Ile130, Phe139, Val150, Pro209, Phe263, Val264, Leu315 and Ile345 form a hydrophobic cavity that accommodates the adenosine moiety of ADP; the ribose group of ADP forms a water molecule-mediated hydrogen bond with Asp269; the adenine group of ADP is coordinated by Gln261 and the main chain atoms of Leu262, Val264 and Tyr267 via a hydrogen bond network ( Fig. 2a ). 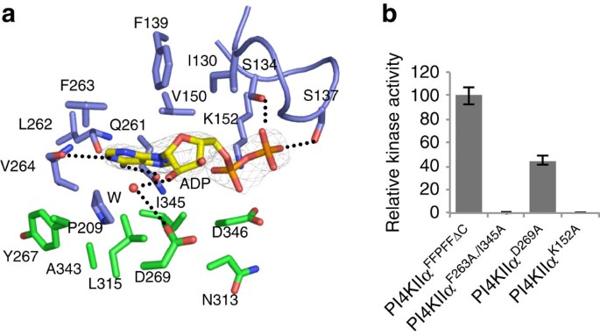Figure 2: Nucleotide-binding pocket of PI4KIIα. (a) Interactions between ADP and PI4KIIα. Residues involved in ADP binding are labelled and shown as stick models with those from the N-lobe coloured in blue and those from the C-lobe coloured in green. A water molecule (W, red) is shown in sphere. The 2Fo-Fc electron density map is shown as a grey mesh and contoured at 1.8σ. Hydrogen bonds are shown as dashed lines. See alsoTable 2. (b) Kinase activities of PI4KIIα variants with mutations at the nucleotide-binding site. Kinase activity was measured in PI/Triton X-100 (0.2%) and normalized by using the activity of PI4KIIαFFPFFDCas 100%. The error bars represent the s.d. from three independent experiments. Figure 2: Nucleotide-binding pocket of PI4KIIα. ( a ) Interactions between ADP and PI4KIIα. Residues involved in ADP binding are labelled and shown as stick models with those from the N-lobe coloured in blue and those from the C-lobe coloured in green. A water molecule (W, red) is shown in sphere. The 2Fo-Fc electron density map is shown as a grey mesh and contoured at 1.8σ. Hydrogen bonds are shown as dashed lines. See also Table 2 . ( b ) Kinase activities of PI4KIIα variants with mutations at the nucleotide-binding site. Kinase activity was measured in PI/Triton X-100 (0.2%) and normalized by using the activity of PI4KIIα FFPFFDC as 100%. The error bars represent the s.d. from three independent experiments. Full size image Next, we compare the structure of ADP-bound PI4KIIα with that of ATP-bound PI3K p110γ (PI3Kγ) ( Table 2 ). Although both kinases have adenosine-binding pockets formed by hydrophobic residues, differences in these residues (from PI4KIIα to PI3Kγ: Ile130 → Met804, Phe139 → Trp812, Val150 → Ile831, Pro209 → Tyr867, Phe263 → Ile881, Leu315 → Met953 and Ala343 → Phe961) generate binding cavities of different shapes and volumes and, therefore, determine the kinases’ specific adenosine-binding affinities. PI4KIIα also has additional interactions with ADP via Gln261 and Asp269. Table 2 Summary and comparison of the important residues and types of interactions for nucleotide binding in PI4KII α and PI3K γ . Full size table To corroborate the above structural analysis, we generated four variants using the palmitoylation mimic mutant PI4KIIα FFPFFΔC ( Supplementary Table 1 ) since this mutant has a higher kinase activity than PI4KIIα SSPSSΔC (ref. 29 ). In comparison with PI4KIIα FFPFFΔC , mutations PI4KIIα F263A/I345A and PI4KIIα K152A inactivate the kinase completely ( Fig. 2b ), and the activity of mutant PI4KIIα D269A is reduced to 44.9%. Structural elements for membrane binding PI4KIIα behaves as an ‘integral’ membrane protein without a transmembrane domain [29] . We utilized a membrane sequential elution assay [29] to study membrane binding of PI4KIIα ( Fig. 3a,b ). Wild-type construct PI4KIIα CCPCC could not be eluted from the membrane by 1M NaCl, but was partially eluted by 0.1 M Na 2 CO 3 and completely eluted by 1.0% Triton X-100, indicating the presence of strong hydrophobic interactions between PI4KIIα and membrane ( Fig. 3a ). Increases in pH or NaCl concentration increased the elution of construct PI4KIIα SSPSSΔC , revealing the contribution of electrostatic interactions ( Fig. 3a ). In addition to the palmitoylation motif, the C-terminal region (454–479) of PI4KIIα is also reported to contribute to membrane binding by hydrophobic interactions [33] . We confirmed this observation ( Fig. 3b ) by comparing the elution behaviours among the constructs PI4KIIα SSPSS , PI4KIIα FFPFF , PI4KIIα SSPSSΔC and PI4KIIα FFPFFΔC ( Supplementary Table 1 ). Deletion of the C-terminal region decreased membrane-binding affinity. The decreased interaction was restored, however, by mutating SSPSS to FFPFF, suggesting that the palmitoylation motif plays a role in membrane binding ( Fig. 3b ). 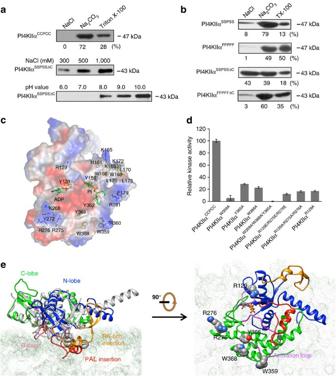Figure 3: Membrane binding of PI4KIIα and its kinase activity. (a,b) Sequential membrane elution assay to evaluate the membrane binding of PI4KIIα variants. (c) The membrane-binding surface of PI4KIIα deduced from the crystallographic packing analysis and mapped with its electrostatic potentials. Blue represents positive charges and red represents negative charges. ADP and the putative PI (seeFig. 4b) are shown as stick models. Residues potentially involved in membrane binding are indicated accordingly. (d) Kinase activities of the PI4KIIα variants. The kinase activity was measured in PI/Triton X-100 (0.2%) and monitored by ADP production. The error bars represent the s.d. from three independent experiments. (e) A representative model of PI4KIIα bound to membrane, obtained from MD simulations. The crystal structure is coloured in grey and the MD structural model is shown with the same scheme ofFig. 1c. The residues evaluated in (d) are indicated accordingly. The simulated membrane is depicted in transparent dots. The left panel is perpendicular to the membrane and the right one is parallel and viewed from the membrane side. Figure 3: Membrane binding of PI4KIIα and its kinase activity. ( a , b ) Sequential membrane elution assay to evaluate the membrane binding of PI4KIIα variants. ( c ) The membrane-binding surface of PI4KIIα deduced from the crystallographic packing analysis and mapped with its electrostatic potentials. Blue represents positive charges and red represents negative charges. ADP and the putative PI (see Fig. 4b ) are shown as stick models. Residues potentially involved in membrane binding are indicated accordingly. ( d ) Kinase activities of the PI4KIIα variants. The kinase activity was measured in PI/Triton X-100 (0.2%) and monitored by ADP production. The error bars represent the s.d. from three independent experiments. ( e ) A representative model of PI4KIIα bound to membrane, obtained from MD simulations. The crystal structure is coloured in grey and the MD structural model is shown with the same scheme of Fig. 1c . The residues evaluated in ( d ) are indicated accordingly. The simulated membrane is depicted in transparent dots. The left panel is perpendicular to the membrane and the right one is parallel and viewed from the membrane side. Full size image By analysing the buried interfaces of PI4KIIα’s crystallographic octamers, we found the potential membrane-binding surface of PI4KIIα. Both octamers A 8 and B 8 involve two tetramers with opposite directions packed together ( Supplementary Fig. 2c,d ). Four bulky hydrophobic residues, Trp359, Tyr362, Tyr365 and Trp368, are located on the plane formed by the packing interface of the tetramers ( Fig. 3c ); the ADP binding pocket and the palmitoylation motif - 174 CCPCC 178 - are also located in this plane. Furthermore, many positively charged residues (Arg129, Arg181, Lys268, Arg275, Arg276 and Arg360) in this plane surround the active site of PI4KIIα. The presence of both hydrophobic and positively charged residues strongly suggests that the tetramer–tetramer interaction interface spans the membrane-binding surface of PI4KIIα. Besides the untraced Trp332 and three embedded Trp273, Trp314 and Trp366, the remaining four Trp residues (Trp359, Trp368, Trp166, Trp169) are exposed to the putative membrane-binding surface of PI4KIIα. The blue shift in the internal fluorescence of Trp when PI4KIIα binds to a liposome ( Supplementary Fig. 5 ) suggests membrane insertion of these Trp residues [36] and, thereby, confirms the membrane-binding function of the above PI4KIIα surface. As an ‘integral’ membrane-binding protein, the kinase activity of PI4KIIα is predicted to depend on its membrane interaction. Perturbation of membrane binding should affect enzymatic activity, as was confirmed in our mutagenesis study. Mutation of hydrophobic residues Trp359, Tyr365 and Trp368 to Ala reduced kinase activity. In addition, abolishing electrostatic interactions with the membrane by mutating positively charged residues Arg129, Arg275 and Arg276 to Ala or Glu had the same effect ( Fig. 3d ). Substitution of Triton X-100 by the ionic detergent Anzergent3-14 significantly upregulated the kinase activity of all tested constructs ( Supplementary Fig. 6 ) since the ‘negatively charged head’ of Anzergent3-14 can enhance electrostatic interactions between PI4KIIα and the surface of the detergent micelle. These results further confirm that the above stated surface of PI4KIIα is involved in membrane association and kinase activity. Considering that the crystal structure of PI4KIIα is in a membrane-free state and that membrane binding might induce conformational change, we carried out MD simulations of the membrane-binding state of PI4KIIα. The initial conformation in the simulations was obtained by placing the crystal structure of PI4KIIα on top of a PI-containing membrane at a distance of 10 Å in one simulation and at a distance of 20 Å in two other simulations ( Supplementary Fig. 7a ). In all three simulations, PI4KIIα was seen to attach to the membrane in 300 ns. Simulations were continued for a total of 1 μs each, resulting in an equilibrated state of membrane-bound PI4KIIα ( Fig. 3e ). The simulation results confirmed that the tetramer–tetramer interface seen in the crystal packing of PI4KIIα coincides with the membrane-binding surface of the kinase ( Fig. 3c ). The palmitoylation and RK-rich insertions exhibited large conformational changes in the simulations ( Fig. 3e , left; Supplementary Movie 1 ) during PI4KIIα’s membrane binding. The amphipathic helix α4 came to lie on the surface of the membrane and the palmitoylation motif inserted deeply into the membrane. Both G-loop and activation loop are involved in membrane binding along with residues R129, R275, R276, W359, Y365 and W368 ( Fig. 3e , right) that are considered important for PI4KIIα’s activity ( Fig. 3d ), as discussed above. Indeed, the MD simulations further confirm the membrane-binding role of all the structural elements deduced from crystallographic and biochemical analysis to interact with the membrane and furnish an atomistic picture of PI4KIIα’s membrane binding. We also performed a 300-ns simulation of PI4KIIα in the absence of membrane as a control ( Supplementary Fig. 7a, #7 ). For this membrane-free simulation, the structure of PI4KIIα is stable without significant conformational changes of palmitoylation and RK-rich insertions and the root mean square deviation relative to the crystal structure stabilized around 2.5 Å, which is a much smaller value than the values seen for simulations in the presence of membrane ( Supplementary Fig. 7a, #1, #2 and #3 ). Putative PI-binding pocket The activation loop of PI3Ks, such as PI3Kγ and Vps34, had been reported to be critical for the binding of PI phosphate [22] , [37] . However, Macphee et al . reported that PI3Ks could phosphorylate PI in both D- and L-form while PI4KIIα has an absolute requirement for the inositol ring to be linked to the glycerol backbone of the lipid through the D-1 position [38] . Therefore, the kinase activity of PI4KIIα is not only related to PI’s inositol head, but also senses the chirality (position D-1) of inositol linked to the glycerol moiety, implying that the binding pocket of PI4KIIα differs from that of the PI3Ks. It is difficult to identify PI-binding pockets of PI4Ks (or PIP 2 -binding pockets of PI3Ks) since binding of the lipid substrate PI (or PIP 2 ) requires the kinase to adopt a membrane-bound conformation, which most likely differs from the crystal form. To go beyond the crystal structure and better understand the PI-binding specificity of PI4KIIα, we analysed further the MD simulation of PI4KIIα in its membrane-bound state. Using the programme HOLLOW [39] , we identified a cavity in PI4KIIα in contact with the membrane surface, proximal to the nucleotide-binding pocket and surrounded by the palmitoylation insertion and activation loop ( Fig. 4a ). We hypothesized this cavity is the PI-binding pocket of PI4KIIα. To test this hypothesis, we carried out three 1-μs MD simulations with palmitoylated PI4KIIα. In one of the simulations, a PI molecule spontaneously bound into this cavity and the binding was stable for the last 500 ns ( Supplementary Movie 2 ). A snapshot of the PI binding PI4KIIα is shown in Fig. 4b . We note that only in one out of three simulations we observed the spontaneous PI binding, which is likely representative for events taking place at much longer (>μs) time scale. 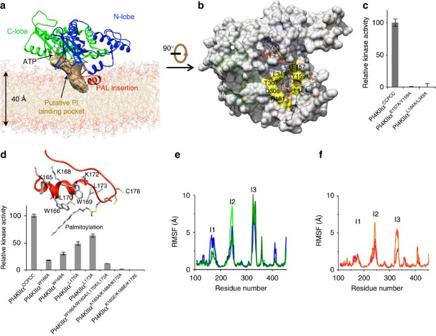Figure 4: Putative PI-binding pocket and palmitoylation insertion-regulated activity of PI4KIIα. (a) Putative PI-binding pocket of PI4KIIα based on molecular dynamics simulations. The cavity surrounded by the palmitoylation insertion and activation loop was computed by using HOLLOW39and rendered in brown surface. (b) Identified important residues for contributing to the PI-binding pocket. These residues are labelled, coloured in yellow and mapped onto the surface of PI4KIIα. The structural model of PI4KIIα including ATP and PI substrates is derived from a snapshot of molecular dynamics simulation. (c) Kinase activities of PI4KIIα variants with mutations at the putative PI-binding pocket. The kinase activity was measured in PI/Triton X-100 (0.2%) and normalized by using the activity of PI4KIIαCCPCCas 100%. All error bars here represent the s.d. from three independent experiments. (d) The kinase activities of PI4KIIα variants with mutations at the amphipathic helix of the palmitoylation insertion. The kinase activity was measured in PI/0.1% Anzergent3-14 and normalized by using the activity of the construct PI4KIIαCCPCCas 100%. The error bars in (c) and (d) represent the s.d. from three independent experiments. (e,f) Conformational fluctuations of PI4KIIα without palmitoylation in (e) and with palmitoylation in (f). Proteins were first aligned to the conformations att=300 ns in each trajectory using backbone atoms of proteins not including three insertions (I1,I2 andI3). The root mean square fluctuation (RMSF) was then calculated using C-alpha atoms of all residues (residue 107 to 453) over the last 700 ns. Blue, green and dark green curves in (e) represent the RMSF statistics from three independent simulations of PI4KIIα without palmitoylation. Orange, red and pink curves in (f) represent three independent simulation of palmitoylated PI4KIIα. Figure 4: Putative PI-binding pocket and palmitoylation insertion-regulated activity of PI4KIIα. ( a ) Putative PI-binding pocket of PI4KIIα based on molecular dynamics simulations. The cavity surrounded by the palmitoylation insertion and activation loop was computed by using HOLLOW [39] and rendered in brown surface. ( b ) Identified important residues for contributing to the PI-binding pocket. These residues are labelled, coloured in yellow and mapped onto the surface of PI4KIIα. The structural model of PI4KIIα including ATP and PI substrates is derived from a snapshot of molecular dynamics simulation. ( c ) Kinase activities of PI4KIIα variants with mutations at the putative PI-binding pocket. The kinase activity was measured in PI/Triton X-100 (0.2%) and normalized by using the activity of PI4KIIα CCPCC as 100%. All error bars here represent the s.d. from three independent experiments. ( d ) The kinase activities of PI4KIIα variants with mutations at the amphipathic helix of the palmitoylation insertion. The kinase activity was measured in PI/0.1% Anzergent3-14 and normalized by using the activity of the construct PI4KIIα CCPCC as 100%. The error bars in ( c ) and ( d ) represent the s.d. from three independent experiments. ( e , f ) Conformational fluctuations of PI4KIIα without palmitoylation in ( e ) and with palmitoylation in ( f ). Proteins were first aligned to the conformations at t= 300 ns in each trajectory using backbone atoms of proteins not including three insertions ( I 1, I 2 and I 3). The root mean square fluctuation (RMSF) was then calculated using C-alpha atoms of all residues (residue 107 to 453) over the last 700 ns. Blue, green and dark green curves in ( e ) represent the RMSF statistics from three independent simulations of PI4KIIα without palmitoylation. Orange, red and pink curves in ( f ) represent three independent simulation of palmitoylated PI4KIIα. Full size image The model of PI4KIIα with PI bound, resulting from MD simulation, shows that both the inositol head group and the glycerol moiety of PI insert into the putative PI-binding pocket, which is lined by residues E157, Y159, R181, L184, T307, D308 and L349 on the palmitoylation insertion and activation loop, respectively ( Fig. 4b ). In order to verify in how far these residues determine the binding specificity for PI’s inositol head group, we carried out a mutagenesis study, in which we perturbed the putative PI-binding pocket by mutating Glu157 and Phe159 to Ala and by mutating Leu184 and Leu349 to Ala. We found that either perturbation could completely diminish the kinase activity of PI4KIIα ( Fig. 4c ). Besides contributing to the PI-binding pocket, the palmitoylation insertion also interacts with the membrane via an amphipathic helix α4. The amphipathic helix α4 not only inserts its bulky hydrophobic residues (Trp166, Trp169, Leu170 and Leu173) into the membrane, but also attracts negatively charged lipid head-groups by electrostatic anchoring via positively charged residues (Lys165, Lys168 and Lys172) ( Figs 3e and 4a,d ). Although this amphipathic helix does not contribute directly to the PI-binding pocket, any perturbation of weakening its membrane interaction by mutating hydrophobic residues to Ala or mutating positively charged residues to Ala/Glu significantly impairs the kinase activity of PI4KIIα ( Fig. 4d ). In addition, we noted that the closer to the PI-binding pocket the mutation site is, the lower the kinase activity of the mutant. These results suggest that the membrane interactions of the amphipathic helix α4 influence the PI binding pocket allosterically and, thereby, modulate PI4KIIα’s activity. Besides the palmitoylation motif (-CCPCC-) [29] , the amphipathic helix α4 is apparently another important element of the palmitoylation insertion that plays a key role in the regulation of PI4KIIα’s activity. The important role of the palmitoylation insertion The possible regulation mechanism via PI4KIIα’s membrane interaction was further investigated based on the MD simulation data ( Fig. 4e,f ; Supplementary Fig. 7 ). We monitored the relative height of PI4KIIα’s centre of mass with respect to the lipid membrane ( Supplementary Fig. 7b ) and the membrane-insertion depth of the palmitoylation insertion (residue 166–179) ( Supplementary Fig. 7c ). It is found that palmitoylation has little effect on the relative height and membrane-insertion depth. However, there is a significant structural fluctuation change as reflected by the root mean square fluctuation of the proteins. With reference to the protein conformation at t =300 ns, in the following 700 ns simulations, PI4KIIα exhibits large conformational fluctuation around three structural insertions, the palmitoylation insertion (I1), RK-rich insertion (I2) and insertion I3. Such large conformational fluctuations were not observed in the membrane-free simulation ( Supplementary Fig. 7d ), suggesting that they originate from PI4KIIα’s interaction with the membrane. In additional, such conformational fluctuations are reduced by~50% for the palmitoylated protein, especially at the palmitoylation insertion region ( Fig. 4e,f ). Based on the analysis of biochemical data ( Fig. 4d ) and MD simulations ( Fig. 4e,f ), we conclude that PI4KIIα’s palmitoylation does not change the strength of its membrane binding significantly, but rather modulates the fluctuations of the protein conformation and, thereby, regulates its kinase activity via tuning the PI-binding pocket. Such conclusion is consistent with our enzymatic study of the non-palmitoylated PI4KIIα CCPCC and palmitoylation-mimic mutant PI4KIIα FFPFF ( Supplementary Fig. 8a ). The upregulated kinase activity of PI4KIIα FFPFF is due to the significantly increased catalysis efficiency (V max ) that is relevant for the stability of the substrate-binding pocket (the energy barrier to overcome in forming the catalytic ternary complex). Therefore, reduced fluctuation due to palmitoylation insertion ( Fig. 4e,f ) would increase the stability of the PI-binding pocket and, thereby, increase catalytic efficiency, resulting in net increase of kinase activity. Our observations suggested the importance of membrane environment for PI4KIIα activity, which was also proposed from previous studies based on the Golgi/endosomal pool [31] . To further verify our observations, we designed an in vitro biochemical assay system by reconstituting PI4KIIα onto liposomes with different lipid compositions. Consistent with our predictions, the presence of 10% cholesterol, which decreased the fluidity and fluctuation of membrane, indeed stimulated higher kinase activities for both PI4KIIα FFPFF and PI4KIIα CCPCC than did the cholesterol-free system ( Supplementary Fig. 8b ). We reported here the first crystal structure in the PI4Ks family, namely PI4KIIα. The structure reveals a distinct nucleotide-binding pocket that is responsible for PI4KIIα insensitivity to PI3Ks’ inhibitors [15] , [16] , [17] and is important for designing specific PI4KIIα’s inhibitors or activators for future therapies of related diseases. Structural comparison, mutagenesis and MD simulations showed that two structural insertions (the palmitoylation insertion and RK-rich insertion) of PI4KIIα are critical for the regulation of PI4KIIα’s membrane binding and kinase activity. The identified putative PI-binding pocket is formed both by activation loop and palmitoylation insertion; pocket conformation is tuned by the nearby palmitoylation motif and amphipathic helix, which become inserted into the membrane when PI4KIIα attaches to the latter. The G-loop from the nucleotide-binding pocket also interacts with the membrane via residue R129 ( Fig. 3e , right). Mutating R129 to Ala results in a significant reduction of PI4KIIα’s kinase activity ( Fig. 3d ). The results suggest that any perturbation of the interaction between PI4KIIα and membrane, such as alteration of the protein ( Figs 3d and 4d ), palmitoylation [28] , [29] , exchanging detergent ( Supplementary Fig. 6 ) and adding cholesterol into the membrane ( Supplementary Fig. 8b ), will affect either the nucleotide binding or PI binding and then modulate the kinase activity of PI4KIIα. In particular, change of the membrane environment via altering lipid composition or through adding specific chemical compounds should regulate the kinase activity of PI4KIIα. Our results are consistent with and provide structural explanations for previous studies of PI4KIIα. Waugh et al . [31] found that tetradeca peptide mastoparan can stimulate activity of PI4KIIα from the Golgi/endosomal pool in a cholesterol dependent manner and suggested that PI4KIIα activity is regulated by changes of the membrane environment. Banerji et al . [32] found that oxysterol-binding protein silencing reduces the cholesterol content of endosome/TGN fractions containing PI4KIIα and then blocks the sterol-sensitive activity of PI4KIIα. Minogue et al . [30] studied intensively the relationship between the kinase activity of PI4KIIα and cholesterol and concluded that cholesterol modulates PI4P synthesis through effects on membrane organization and enzyme diffusion. Min Suk Kang et al . [14] recently found ginsenoside (20S)Rg3, a sterol-like compound, can lower the level of β-amyloid peptide via increasing the activity of PI4KIIα in neurons and they suggested that (20S)Rg3 modulates PI4KIIα in a manner similar to cholesterol-dependent regulation of PI4KIIα activity and PI4P production. Altogether, our current study has provided molecular insight into how the kinase activity of PI4KIIα can be regulated via changing membrane organization. Plasmids and materials The original plasmid of full-length human PI4KIIα was a kind gift of Shane Minogue (University College London) [7] . PI was purchased from Sigma-Aldrich (US, Cat. No. P6636), and an ADP-Glo kinase kit was purchased from Promega (US, Cat. No. V9102). Protein expression and purification The construct PI4KIIα SSPSSΔC (see Supplementary Table 1 ) was expressed as a GST fusion protein in E. coli BL21-CodonPlus (DE3). Cells were grown at 37 °C until the OD 600 reached 1.0 and then induced by 0.3 mM isopropyl β- D -thiogalactoside at 16 °C for 18 h. Cells were then harvested and re-suspended in buffer containing 1% LDAO, 50 mM Hepes, pH 7.5, 1 M NaCl, 2 mM DTT, 10 mM MgCl 2 , 1 mM phenylmethylsulfonyl fluoride and 1 mg ml −1 lysozyme. Cell suspensions were homogenized with a high pressure cell disruptor (JN BIO) at 30,000 psi. Cell debris was removed by centrifugation at 120,000 g for 40 min. Proteins were purified using a GST-affinity column (GE Healthcare). The GST tag was cleaved overnight at 4 °C with PreScission protease (GE Healthcare) in buffer containing 50 mM Hepes, pH 7.5, 300 mM NaCl, and 2 mM DTT. The cleaved proteins were desalted and then applied to the HiTrap Heparin column (GE Healthcare) that was equilibrated with buffer A containing 100 mM glycine pH9.5, 50 mM NaCl, 2 mM MgCl 2 and 2 mM DTT. Elution was carried out with a gradient of NaCl concentration from 50–500 mM. The peak was eluted at~250 mM NaCl. Then the collected proteins were desalted again before loading onto a Mono Q column (GE Healthcare) that was pre-equilibrated with buffer A. Elution was carried out with a gradient of NaCl concentration from 50–500 mM. The peak was eluted at~220 mM NaCl. The purified proteins were concentrated to 30 mg ml −1 with the buffer changing to 25 mM Tris–HCl, pH 8.5, 150 mM NaCl by ultra-filtration using Amicon Ultra-4 centrifugal filters (Millipore). A selenomethioninyl derivative of PI4KIIα SSPSSΔC (Se- PI4KIIα SSPSSΔC ) was prepared as described previously [40] . In brief, the expression vector containing PI4KIIα SSPSSΔC was transformed into the methionine auxotroph E. coli B834 strain (Novagen). The cells were grown in M9 medium supplemented with YNB medium, 0.05 g ml −1 glucose, 2 mM MgSO 4 , 0.1 mM CaCl 2 and 30 mg l −1 of L-selenomethionine (Sigma). Se-PI4KIIα SSPSSΔC was purified in the same way as described above for PI4KIIα SSPSSΔC . All the variants in mutagenesis studies on PI4KIIα were generated using a standard PCR-based protocol, and were expressed and purified in the same way as the construct PI4KIIα SSPSSΔC . Construct PI4KIIα EΔN93 was expressed in Hi5 insect cells using a baculovirus expression system (Bac-to-Bac; Invitrogen). The membrane was prepared from the PI4KIIα EΔN93 -expressing Hi5 insect cells by differential centrifugation and homogenized in buffer containing 50 mM Hepes, pH 7.5, 0.3 M NaCl, 2 mM DTT, 2 mM MgCl 2 , 1 mM phenylmethylsulfonyl fluoride and antiprotease cocktail (Roche; Brussels, Belgium). The membrane suspension was stirred on ice and Triton X-100 was added slowly to a final concentration of 1%. After 30 min incubation, the solution was centrifuged for 30 min at 150,000 g to collect the supernatant. PI4KIIα EΔN93 was then purified according to the same protocol as used for construct PI4KIIα SSPSSΔC . The protein concentration was determined using the BCA (bicinchoninic acid) method [41] with bovine serum albumin as standard. SDS–PAGE was performed on 12% polyacrylamide gels. Crystallization and data collection Purified PI4KIIα SSPSSΔC (~30 mg ml −1 ) was diluted with a buffer containing 25 mM HEPES, pH 7.5, 150 mM NaCl, 1 mM DTT and 20 mM MgCl 2 to a final concentration of 4 mg ml −1 . The detergent hexaethylene glycol monooctyl ether (C 8 E 6 ; Anatrace) was added to a final concentration of 20 mM. After incubation on ice for 30 min, the protein solution was centrifuged at 15000 g for 30 min. The pellet was discarded and the supernatant was collected for crystallization. Crystals of PI4KIIα SSPSSΔC were grown by the hanging-drop vapour diffusion method at 293 K by mixing 1 μl of protein solution with an equal volume of reservoir solution containing 0.1 M citric acid, pH 5.8, 150 mM NaCl and 18% PEG400. Data collection and structure determination Crystals of PI4KIIα SSPSSΔC were flash-frozen in liquid nitrogen. The diffraction data were collected at 100 K by using the beamline BL17U of SSRF (Shanghai Synchrotron Radiation Facility) and processed with HKL2000 (ref. 42 ). The crystals of PI4KIIα SSPSSΔC belong to the space group I422. Single anomalous diffraction (SAD) data of the PI4KIIα SSPSSΔC selenomethionine derivatives was collected at 3.2 Å resolution with the wavelength of 0.9791 Å. Selenium atoms were determined with the SHELXD [43] programme in HKL2MAP [44] . Phases were calculated and refined with SOLVE [45] and RESOLVE [46] . An initial model was built using COOT [47] and further refined using REFMAC5 (ref. 48 ). Diffraction data for the native PI4KIIα SSPSSΔC crystal was collected with the wavelength of 0.9793 Å and processed to 2.95 Å resolution. Its crystal structure was determined by molecular replacement using PHASER [49] and further refined using REFMAC5 (ref. 48 ). Stereochemistry of the final structures was validated with PROCHECK [50] and MolProbity [51] . The statistics for data processing and structure refinements are summarized in Table 1 . Proteoliposome preparation Purified PI4KIIα variants were reconstituted in liposomal membranes using a detergent removal method [52] . Lipid mixtures (60% phosphatidylinositol, 20% phosphatidylserine, 10% cholesterol and 10% phosphatidyl acid) were co-dissolved in chloroform/methanol and then dried in a clean tube overnight under vacuum. Lipid films were rehydrated at 37 °C in buffer containing 25 mM HEPES, pH 7.4, 150 mM NaCl and 2 mM MgCl 2 . The lipid solution was frozen in liquid nitrogen and thawed in air five times before being extruded through a 100 nm pore filter (Avanti Polar Lipids) to produce liposomes with a diameter of 100 nm. Final lipid concentration was ~2 mg ml −1 . To reconstitute purified protein in the liposomes, purified PI4KIIα variants were mixed with liposomes at a protein:lipid ratio of 1:20 in the presence of 0.2% Triton X-100. The mixture was incubated for 1 h at 4 °C before treating with SM-2 Bio-Beads (Bio-Rad) to absorb the detergent. 270 mg of wet SM-2 Bio-Beads, pretreated as described by Levy et al . [53] , were added per ml protein–lipid–detergent mixture. Absorption treatments were recorded after 45 min agitation at 4 °C and repeated three times. Finally, 500 mg of SM-2 Bio-Beads were added to completely remove detergent by shaking the solution gently overnight at 4 °C. Alternatively, the mixture was dialyzed overnight against the buffer, 25 mM HEPES, pH 7.4, 150 mM NaCl and 2 mM MgCl 2 , to remove Triton X-100. Co-sedimentation assay was used to verify the binding of PI4KIIα to the liposome membrane. Kinase activity assay PI4KIIα activity was determined by measuring ADP generation using an ADP-Glo kinase kit (Promega) as previously described [54] . Briefly, 1 μg protein in a kinase buffer containing 20 mM Tris, pH 7.5, 150 mM NaCl, 0.2% Triton X-100 (or 0.1% Anzergent 3–14), 1 mM EDTA and 20 mM MgCl 2 was used in this assay. PI dissolved in chloroform was dried using nitrogen, resuspended to 7 mM in the above kinase buffer and then sonicated for 30 min before use. Protein 1 μl (1 mg ml −1 ) was mixed with 7 μl kinase buffer and 10 μl PI micelles. The kinase reaction was initiated by adding 2 μl ATP (10 mM) and carried out at room temperature (RT). All reactions were repeated three times and were controlled with blank reactions that lacked PI. Reactions were stopped by addition of 20 μl ADP-Glo reagent (Promega). After 60 min incubation at RT, 40 μl of Kinase Detection Reagent (Promega) was added and the mixture was incubated for another 60 min at RT. The fluorescence signal of the mixture was recorded on a Luminescence Spectrometer set to a sensitivity of 30%. Membrane elution assay Bacteria overexpressing PI4KIIα and its mutants were homogenized in a solution containing 50 mM HEPES, pH 7.5, 150 mM NaCl, 2 mM MgCl 2 , 2 mM DTT, 10 μg ml −1 RNaseA and 1 mg ml −1 lysozyme, and then disrupted with a high pressure disruptor (JN BIO) at 30,000 psi. The lysate was centrifuged at 17,000 g for 20 min. The supernatant was further centrifuged at 150,000 g for 2 h to collect the membrane fraction. Membrane pellets were homogenized in a solution containing 20 mM Tris–HCl, pH 7.5, 1 M NaCl, and 1 mM EDTA, and then centrifuged at 200,000 g for 15 min. The resulting supernatant contained weakly membrane-bound proteins. Pellets were further homogenized in 0.1 M sodium carbonate (pH 11.0) and centrifuged at 200,000 g for 15 min to obtain tightly bound peripheral membrane proteins (supernatant fraction). Finally, new pellets were homogenized again in 1.0% Triton X-100 and centrifuged as described above to obtain the integral membrane proteins (supernatant fraction) [29] . Equal amounts of each supernatant fraction were analysed by western blotting with anti-GST antibodies (Novagen) in a dilution of 1:10,000 that were followed by HRP-labelled secondary antibodies. An enhanced chemiluminescence kit (Pierce) was used to visualize the target proteins. Uncropped images of blots are shown in Supplementary Fig. 9 . The band intensity was quantified using Scion Image Analysis Software (Scion, USA). PI4KIIα internal tryptophan fluorescence PI4KIIα internal fluorescence measurements were performed on a Hitachi F-4500 Fluorescence Spectrophotometer at 20.0±0.1 °C. The excitation wavelength was set to 295 nm and emission was scanned from 315 nm to 400 nm at a scan speed of 60 nm min −1 . The excitation and emission spectral slits were set to 10 nm. Each sample was scanned three times and averaged data are presented. MD simulation The atomic coordinates of PI4KIIa were taken from the crystal structure reported in the current study. Lipid membranes, composed of 50% dioleoylphosphatidylcholine lipids (neutral), 33% dioleoylphosphatidylserine lipids (−1e charged) and 17% phosphoinositol, were assumed in all simulations. PI4KIIa without palmitoylation was placed on top of the resulting lipid patch with no initial contacts to the membrane. The palmitoylated PI4KIIa was modelled based on the equilibrated structure of PI4KIIa at the end of a 1 μs simulation of PI4KIIa without palmitoylation. ATP was modelled to the position of the ADP molecule resolved in the crystal structure. Sodium and chloride ions were added to neutralize the simulated systems and to reach an ion concentration of 150 mM; the TIP3P water model [55] was used for solvation. In the simulations of palmitoylated PI4KIIa, the palmitoylation group was added to residue CYS175. Parameters for palmitoylated CYS175 were obtained by using the force field toolkit [56] . The resulting models contained ~270 k atoms. Details of the simulation can be found in Supplementary Note 1 . All simulations were performed using NAMD 2.9 (ref. 57 ) and were analysed using VMD [58] . How to cite this article : Zhou, Q. et al . Molecular insights into the membrane-associated phosphatidylinositol 4-kinase IIα. Nat. Commun. 5:3552 doi: 10.1038/ncomms4552 (2014). Accession codes : The atomic coordinates and the structure factor files for the crystal structures of the catalytic domain of PI4KIIa bound with ADP and its selenomethionine derivative are deposited in the Protein Data Bank with the accession numbers 4HNE and 4HND , respectively.